mGlu5 receptors regulate synaptic sumoylation via a transient PKC-dependent diffusional trapping of Ubc9 into spines Sumoylation plays important roles in the modulation of protein function, neurotransmission and plasticity, but the mechanisms regulating this post-translational system in neurons remain largely unknown. Here we demonstrate that the synaptic diffusion of Ubc9, the sole conjugating enzyme of the sumoylation pathway, is regulated by synaptic activity. We use restricted photobleaching/photoconversion of individual hippocampal spines to measure the diffusion properties of Ubc9 and show that it is regulated through an mGlu5R-dependent signalling pathway. Increasing synaptic activity with a GABA A receptor antagonist or directly activating mGlu5R increases the synaptic residency time of Ubc9 via a Gα q /PLC/Ca 2+ /PKC cascade. This activation promotes a transient synaptic trapping of Ubc9 through a PKC phosphorylation-dependent increase of Ubc9 recognition to phosphorylated substrates and consequently leads to the modulation of synaptic sumoylation. Our data demonstrate that Ubc9 diffusion is subject to activity-dependent regulatory processes and provide a mechanism for the dynamic changes in sumoylation occurring during synaptic transmission. Neurons are specialized cells, which connect through synapses for rapid information transfer in the brain. The efficiency of synaptic transmission largely depends on the correct targeting and arrangement of complex protein networks on both sides of the synapse. These processes are almost always regulated by post-translational modifications such as phosphorylation or ubiquitination [1] . Sumoylation is emerging as a potent post-translational mechanism important for the regulation of synaptic transmission and plasticity [2] , [3] , [4] . The proper functioning of such modifications requires a rigorous spatial and temporal control of the associated enzymatic machinery. However, the regulatory mechanisms of the sumoylation machinery are still largely unknown, especially at synapses. Sumoylation consists in the covalent binding of the small ubiquitin-like modifier peptide SUMO to specific lysine residues of target proteins [5] , [6] . Three SUMO paralogues have been identified so far. Protein sumoylation is mediated through a specific enzymatic cascade. Matured SUMO moieties are activated by the E1-activating complex. Then, SUMO is transferred onto the E2 Ubc9, the sole conjugating enzyme of the system. The covalent SUMO attachment to lysine residues requires the binding of Ubc9 to target proteins through its C93-containing catalytic domain [7] , [8] and, either directly or in conjunction with one of the E3 enzymes Ubc9, catalyses SUMO conjugation to substrate proteins [7] , [8] . Many target proteins bear a phospho-dependent sumoylation motif (PDSM) [9] . The phosphorylation of this motif leads to an increase in the binding of Ubc9 to phosphorylated target proteins compared with their unmodified counterparts [9] , [10] . Importantly, sumoylation is a reversible process through the action of specific isopeptidases called sentrin-specific proteases [11] . Molecular consequences of sumoylation are multiple. Sumoylation may mask protein–protein interaction sites, create new binding interfaces or lead to conformational changes. Another emerging role for sumoylation in the central nervous system is the propensity to regulate protein aggregation [3] , [12] , [13] , [14] . Sumoylation can also directly impact on other post-translational modifications. For instance, sumoylation and ubiquitination processes can compete to modify the same lysine residue to dynamically control protein stability [15] , [16] . In neurons, sumoylation influences various aspects of neuronal activity [2] , [3] and modifies the stability and activity of several transcription factors known to regulate neuronal morphogenesis and postsynaptic differentiation [10] , [17] , [18] , [19] . We reported the presence of multiple unidentified sumoylation substrates at synapses [20] . Since then, several studies including ours, reported that cytosolic and integral plasma membrane proteins important for synaptic transmission and plasticity are sumoylated, thereby modulating their stability, subcellular targeting, trafficking or interacting properties [12] , [13] , [20] , [21] , [22] , [23] , [24] , [25] . Although sumoylation has impacts on key neuronal processes, the regulatory mechanisms of this enzymatic system at synapses are still unknown. Therefore, investigating the spatiotemporal regulation of the SUMO system in the spines is of particular interest to better understand the synaptic function of sumoylation. We reported the developmental regulation of the SUMO system in the rat brain and showed an enrichment of sumoylation enzymes at synapses during neuronal maturation [26] . We further demonstrated that neuronal depolarization evokes a redistribution of the endogenous sumoylation machinery in spines, indicating that sumoylation is dynamically regulated by neuronal activity [27] . Here we characterize the activity-dependent synaptic diffusion of Ubc9, the sole conjugating enzyme of the SUMO system, using a live-imaging approach on rat hippocampal neurons. We demonstrate that Ubc9 is highly mobile in neurons and that its synapto-dendritic mobility is not regulated by N -methyl- D -aspartate receptors (NMDARs) but through a signalling cascade downstream of the activation of metabotropic glutamate 5 receptors (mGlu5R). Activation of mGlu5R leads to an increased synaptic residency time for the active form of Ubc9. This mGlu5R-induced diffusional trapping is prevented when the signalling pathway downstream of Gα q proteins, but not downstream of Gα i , is blocked. We further show that the pharmacological blocking of phospholipase C (PLC) activity, calcium influx from L-type voltage-dependent calcium channels (L-VDCCs) or from internal stores or protein kinase C (PKC) activity abolishes the mGlu5R-dependent synaptic regulation of Ubc9. Interestingly, the transient diffusional trapping observed in mGlu5R- or phorbol 12-myristate 13-acetate (PMA)-activated spines is lost with the catalytically inactive and substrate-binding-deficient Ubc9-C93S mutant or with the Ubc9-K65A enzyme, which, contrary to the WT Ubc9, loses its ability to preferentially recognize phosphorylated substrates. Altogether, our data demonstrate that the transient diffusional trapping of Ubc9 measured in mGlu5R-activated spines results from an increased Ubc9 recognition to PKC-phosphorylated synaptic substrate proteins, ultimately promoting synaptic sumoylation. The diffusion of Ubc9 is regulated by synaptic activity To examine whether neuronal activity regulates the synaptic diffusion of the sumoylation machinery, we expressed the wild-type (WT) form of the SUMO-conjugating enzyme Ubc9 fused in frame to the green fluorescent protein carboxy terminus (GFP-Ubc9) in cultured hippocampal neurons ( Fig. 1 ). As previously demonstrated for the endogenous enzyme, we found high levels of GFP-Ubc9 fluorescence in the nucleus, indicating that the GFP tag does not impair the nucleocytoplasmic transport of Ubc9. GFP-Ubc9 fluorescence was also distributed throughout the dendrites where it displayed a clear synaptic distribution in addition to lower levels of diffuse staining in the shaft ( Fig. 1a ). We next evaluated whether the GFP tag would prevent Ubc9 activity. We co-expressed GFP-Ubc9 or its inactive C93S mutant with mCherry-SUMO1 or mCherry-SUMO2 in COS7 cells ( Supplementary Fig. 1 ). We showed that contrary to the Ubc9-C93S inactive mutant, GFP-Ubc9 was active and able to increase protein sumoylation levels when co-expressed with mCherry-SUMOs. Together, these findings indicated that GFP-Ubc9 is active with a subcellular localization comparable to the neuronal distribution reported for the endogenous enzyme [20] , [26] . 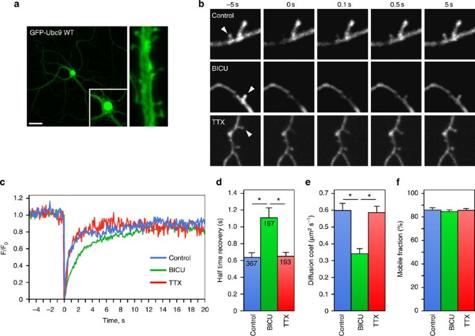Figure 1: Activity-dependent synaptic diffusion of GFP-Ubc9 in hippocampal neurons. (a) Representative image of a 20 daysin vitro(DIV) rat hippocampal neuron expressing GFP-Ubc9. Note that GFP-Ubc9 is mainly localized within the nucleus (inset). GFP-Ubc9 fluorescence is also distributed in dendrites and spines. Scale bar, 20 μm. (b) Images from representative GFP-Ubc9 FRAP experimental time course in basal (Ctrl), bicuculline (BICU, 10 μM) or tetrodotoxin (TTX, 2 μM)-treated conditions. (c) Normalized FRAP curves from spines inbshowing recovery of GFP-Ubc9 fluorescence after photobleaching over the course of 20 s in basal control, enhanced (BICU) or decreased (TTX) synaptic activity. Summary histograms of FRAP experiments showing the means (±s.e.m.) of half-time of recovery (d), diffusion coefficients (e) and mobile fractions (f) from the number of bleached spines indicated on the bars (d). (d,e) *P=0.001; one-way analysis of variance. Figure 1: Activity-dependent synaptic diffusion of GFP-Ubc9 in hippocampal neurons. ( a ) Representative image of a 20 days in vitro (DIV) rat hippocampal neuron expressing GFP-Ubc9. Note that GFP-Ubc9 is mainly localized within the nucleus (inset). GFP-Ubc9 fluorescence is also distributed in dendrites and spines. Scale bar, 20 μm. ( b ) Images from representative GFP-Ubc9 FRAP experimental time course in basal (Ctrl), bicuculline (BICU, 10 μM) or tetrodotoxin (TTX, 2 μM)-treated conditions. ( c ) Normalized FRAP curves from spines in b showing recovery of GFP-Ubc9 fluorescence after photobleaching over the course of 20 s in basal control, enhanced (BICU) or decreased (TTX) synaptic activity. Summary histograms of FRAP experiments showing the means (±s.e.m.) of half-time of recovery ( d ), diffusion coefficients ( e ) and mobile fractions ( f ) from the number of bleached spines indicated on the bars ( d ). ( d , e ) * P =0.001; one-way analysis of variance. Full size image To assess the synaptic transport of Ubc9 in real time, we performed restricted photobleaching experiments to measure the fluorescence recovery after photobleaching (FRAP) of individual spines from GFP-Ubc9-expressing neurons ( Fig. 1b–f ). To quantitatively measure Ubc9 diffusion in spines, FRAP data were individually fitted with a single-phase exponential function to obtain values for the mobile fraction and the rate of fluorescence recovery (half-time of recovery; see the Methods section for details). The mobile fraction is the proportion of Ubc9 in the bleached spine that exchanged with unbleached Ubc9 from the dendritic shaft over the time course of the experiment. In absence of stimulation, there was only a small fraction of immobile Ubc9 in spines with ~85% recovery of the initial fluorescence, indicating that bleached GFP-Ubc9 were dynamically exchanged with fluorescent GFP-Ubc9 from the shaft in resting conditions. In resting neurons, the rate of GFP-Ubc9 fluorescence recovery in spines was 0.63 s with a diffusion coefficient of 0.59 μm 2 s −1 ( Fig. 1b–f ). Blocking synaptic activity with the Na + channel blocker tetrodotoxin (TTX) did not have an impact on the diffusion of Ubc9 in spines with values obtained for TTX-treated neurons, similar to those measured in control conditions. Interestingly, increasing synaptic activity by blocking inhibitory GABA A receptors with bicuculline did not affect the ratio of mobile GFP-Ubc9 molecules ( Fig. 1f ) but significantly increased the half-time of GFP-Ubc9 fluorescence recovery ( Fig. 1d ; Control, 0.63±0.05 s; Bicu, 1.1±0.12 s, means±s.e.m.). The direct consequence of this effect is the concomitant decrease in GFP-Ubc9 diffusion coefficient in spines from bicuculline-treated neurons ( Fig. 1e ; Control, 0.59±0.05 μm 2 s −1 ; Bicu, 0.33±0.02 μm 2 s −1 , means±s.e.m.). The fact that the mobile fraction of GFP-Ubc9 remains unaffected in stimulated conditions concurrently to a delayed exchange of the enzyme between the shaft and the spine imply that there is an increase in the synaptic residency time of Ubc9 in activated neurons. We also showed that in contrast to GFP-Ubc9, the synaptic diffusion of free diffusing GFP molecules in spines was not regulated by activity ( Supplementary Fig. 2 ). Ubc9 diffusion is not regulated via NMDAR activation Cytosolic proteins such as the Ca 2+ /calmodulin-dependent protein kinase II or the proteasome subunit Rpt1 are targeted to spines in activated cells predominantly via activation of NMDARs [28] , [29] . We therefore examined whether the increased synaptic residency time of Ubc9 measured in bicuculline-treated neurons was sensitive to NMDAR inhibition ( Fig. 2 ). We performed synaptic FRAP experiments on GFP-Ubc9 expressing neurons and the recovery curves were recorded under bicuculline treatment in the presence of the NMDAR antagonist D-AP5. Inhibition of NMDAR with D-AP5 did not modify the decrease in the rate of GFP-Ubc9 fluorescence recovery when co-incubated with bicuculline ( Fig. 2 ), indicating that the regulation of Ubc9 diffusion in spines is independent of NMDAR activation. 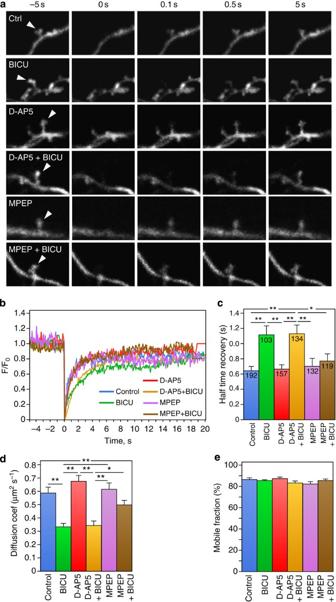Figure 2: mGlu5R-dependent, NMDAR-independent synaptic regulation of Ubc9 diffusion. (a) Sequential images from GFP-Ubc9 FRAP experiments in individual spine (arrowheads). The NMDA receptor antagonist D-AP5 (50 μM) or the specific mGlu5R antagonist MPEP (30 μM) were tested in combination with the GABAAreceptor antagonist bicuculline (10 μM) to determine the involvement of NMDA and mGlu receptors on Ubc9 diffusion. (b) Normalized FRAP curves from spines inashowing recovery of GFP-Ubc9 fluorescence after photobleaching over the time course of the experiment in bicuculline-treated cells. Histograms of FRAP experiments showing the means (±s.e.m.) of half-time of fluorescence recovery (c), diffusion coefficients (d) and mobile fractions (e) from the number of bleached spines indicated on the bars (c). One-way analysis of variance was performed with a Newman–Keuls post test for multiple comparison data sets. (c) **P=0.001 compared with Ctrl, D-AP5, MPEP; *P<0.01 compared with BICU, D-AP5+BICU; (d) **P=0.001 compared with Ctrl, D-AP5, MPEP; *P<0.01 compared with BICU, D-AP5+BICU. Figure 2: mGlu5R-dependent, NMDAR-independent synaptic regulation of Ubc9 diffusion. ( a ) Sequential images from GFP-Ubc9 FRAP experiments in individual spine (arrowheads). The NMDA receptor antagonist D-AP5 (50 μM) or the specific mGlu5R antagonist MPEP (30 μM) were tested in combination with the GABA A receptor antagonist bicuculline (10 μM) to determine the involvement of NMDA and mGlu receptors on Ubc9 diffusion. ( b ) Normalized FRAP curves from spines in a showing recovery of GFP-Ubc9 fluorescence after photobleaching over the time course of the experiment in bicuculline-treated cells. Histograms of FRAP experiments showing the means (±s.e.m.) of half-time of fluorescence recovery ( c ), diffusion coefficients ( d ) and mobile fractions ( e ) from the number of bleached spines indicated on the bars ( c ). One-way analysis of variance was performed with a Newman–Keuls post test for multiple comparison data sets. ( c ) ** P =0.001 compared with Ctrl, D-AP5, MPEP; * P <0.01 compared with BICU, D-AP5+BICU; ( d ) ** P =0.001 compared with Ctrl, D-AP5, MPEP; * P <0.01 compared with BICU, D-AP5+BICU. Full size image Ubc9 diffusion is regulated via an mGlu5R-dependent pathway Activation of metabotropic glutamate receptors (mGluRs) results in diverse actions on neuronal excitability, synaptic transmission and plasticity by modulating the activity of a variety of ion channels and regulatory proteins [30] , [31] . We therefore assessed whether mGluRs are involved in the regulation of Ubc9 diffusion in activated spines ( Fig. 2 ). We showed that preincubation of bicuculline-activated neurons with the specific mGlu5R antagonist 2-methyl-6-(phenylethynyl)pyridine (MPEP) occluded the increase in the half-time of fluorescence recovery ( Fig. 2b,c ; Bicu, 1.1±0.12 s; Bicu+MPEP, 0.70±0.1 s, means±s.e.m.) and the subsequent decrease in Ubc9 diffusion coefficient in activated neurons ( Fig. 2d ; Bicu, 0.33±0.02 μm 2 s −1 ; Bicu+MPEP, 0.50±0.03 μm 2 s −1 , means±s.e.m. ), while it showed no effect on its own on control non-stimulated cells. Mobile fractions were not modified by the treatments ( Fig. 2e ). Our data therefore suggest that the activation of mGlu5R is involved in the synaptic regulation of Ubc9 diffusion. To test whether a direct activation of mGlu5R is required to regulate the synaptic diffusion of Ubc9, GFP-Ubc9-expressing neurons were stimulated with the specific group I mGluR agonist 3,5-dihydroxyphenylglycine (DHPG) and GFP-Ubc9-labelled spines were photobleached during the treatment ( Fig. 3a–e ). Interestingly, although the mobile fraction was unaffected by the stimulation, there was an increase in the half time of fluorescence recovery ( Fig. 3c ; Control, 0.69±0.04 s; DHPG, 1.02±0.05 s, means±s.e.m.) with the concurrent decrease in the diffusion coefficient values ( Fig. 3d ; Control, 0.52±0.02 μm 2 s −1 ; DHPG, 0.34±0.03 μm 2 s −1 , means±s.e.m.). This decreased synaptic diffusion of Ubc9 in DHPG condition was prevented when neurons were co-incubated with the specific mGlu5R antagonist MPEP ( Fig. 3a–d ). As the mobile fraction is unmodified by the mGlu5R activation ( Fig. 3e ), it implies that there is no significant accumulation of Ubc9 into spines. Consistently, although there was only a small increase in synaptic GFP-Ubc9 fluorescence during DHPG treatment, we did not detect any modifications in endogenous synaptic Ubc9 immunoreactivity in mGlu5R-activated neurons ( Supplementary Fig. 3 ). Altogether, our data indicate that mGlu5R activation dynamically regulates the synapto-dendritic diffusion of Ubc9. 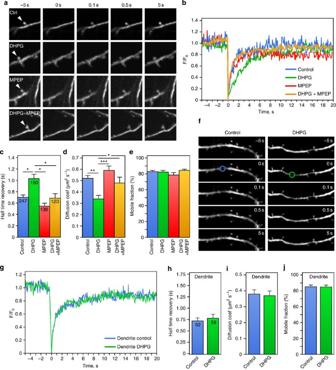Figure 3: mGlu5R-dependent regulation of Ubc9 diffusion at hippocampal synapses. (a) Images from representative GFP-Ubc9 FRAP experimental time course in basal (Ctrl), DHPG, MPEP or DHPG+MPEP conditions. (b) Normalized curves from spines inashowing recovery of GFP-Ubc9 fluorescence after photobleaching over the course of the experiments. Summary histograms of FRAP experiments in panelashowing the means (±s.e.m.) of half-time of fluorescence recovery (c), diffusion coefficients (d) and mobile fractions (e) from the number of bleached spines indicated on the bars (c). (c) *P=0.001; (d) ***P=0.001, **P<0.01, *P<0.05. Images (f) or normalized curves (g) from representative FRAP experiments performed on dendrites of GFP-Ubc9-expressing neurons in basal and DHPG-stimulated conditions. Histograms showing the means (±s.e.m.) of half-time of recovery (h), diffusion coefficients (i) and mobile fractions (j) from the number of bleached dendritic areas indicated on the bars (h). Photobleached GFP-Ubc9 molecules in the shaft were similarly exchanged for fluorescent enzymes in basal and DHPG conditions. Figure 3: mGlu5R-dependent regulation of Ubc9 diffusion at hippocampal synapses. ( a ) Images from representative GFP-Ubc9 FRAP experimental time course in basal (Ctrl), DHPG, MPEP or DHPG+MPEP conditions. ( b ) Normalized curves from spines in a showing recovery of GFP-Ubc9 fluorescence after photobleaching over the course of the experiments. Summary histograms of FRAP experiments in panel a showing the means (±s.e.m.) of half-time of fluorescence recovery ( c ), diffusion coefficients ( d ) and mobile fractions ( e ) from the number of bleached spines indicated on the bars ( c ). ( c ) * P =0.001; ( d ) *** P =0.001, ** P <0.01, * P <0.05. Images ( f ) or normalized curves ( g ) from representative FRAP experiments performed on dendrites of GFP-Ubc9-expressing neurons in basal and DHPG-stimulated conditions. Histograms showing the means (±s.e.m.) of half-time of recovery ( h ), diffusion coefficients ( i ) and mobile fractions ( j ) from the number of bleached dendritic areas indicated on the bars ( h ). Photobleached GFP-Ubc9 molecules in the shaft were similarly exchanged for fluorescent enzymes in basal and DHPG conditions. Full size image The mGlu5R-dependent Ubc9 diffusion is restricted to spines We then asked whether this mGlu5R-dependent regulation of Ubc9 diffusion could be specifically restricted to the synaptic area. We measured the diffusion properties of GFP-Ubc9 in dendrites ( Fig. 3f–j ). In marked contrast to the data obtained on spines, DHPG stimulation led to Ubc9 diffusion parameters in dendrites similar to those measured in non-stimulated neurons with no modification in the rate of GFP-Ubc9 fluorescence recovery ( Fig. 3f–j ), indicating that the mGlu5R-dependent regulation of Ubc9 diffusion is restricted to spines. mGlu5R-dependent diffusional trapping of Ubc9 into spine To confirm that the increased synaptic residency time of Ubc9 in activated neurons results from a brief retention of Ubc9 into spines, we designed experiments in which we could directly visualize the synaptic exit of Ubc9. To perform these experiments, we swapped the GFP from GFP-Ubc9 for the green-to-red photoactivatable Dendra2 (refs 32 , 33 ) protein (Dendra2-Ubc9). Using time-lapse microscopy, we first visualized the loss of the red photoconverted Dendra2-Ubc9 fluorescence from the spine head in basal condition ( Fig. 4 ). We compared the half-time of the red fluorescence decrease from two successive photoconversion events on the same spine (paired recordings) and showed that consecutive photoactivations do not affect the exit rate of Dendra2-Ubc9 in control conditions ( Fig. 4b–d ). In marked contrast, a 10-min mGlu5R stimulation before the second photoconversion led to a significant delay in the exit rate of the red photoconverted fluorescence from the spines (Pre-DHPG, 1.63±0.16 s; post-DHPG, 2.78±0.26 s, means±s.e.m. ; Fig. 4c–e ), further confirming our initial observation using FRAP that mGlu5R activation regulates the synapto-dendritic diffusion of Ubc9. 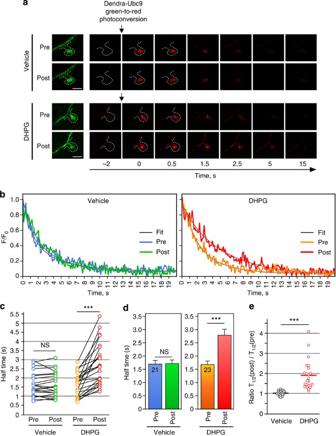Figure 4: mGlu5R activation promotes a transient diffusional trapping of Ubc9 in spines. (a) Time-lapse series of confocal images of photoconverted Dendra2-Ubc9 red fluorescence in spines in control and mGlu5R-stimulated conditions. Images of spine before Dendra2-Ubc9 photoconversion are shown in green (left). Following the first synaptic green-to-red photoconversion, neurons were incubated with control solution (vehicle) or with DHPG (50 μM) for 10 min and spines were photoconverted a second time. The red photoconverted fluorescence was then monitored as described in the Methods section. Scale bar, 1 μm. (b) Representative sample paired recording traces of normalized fluorescence from photoconverted Dendra2-Ubc9 in individual spines before (pre) and after mGlu5R activation (post) as shown ina. The thin traces (black) represent the corresponding fits. (c) Scatter plots of computed half-time of photoconverted Dendra2-Ubc9 fluorescence diffusion in spines pre- and post-DHPG application. Pairedt-test: vehicle,n=21; NS, not significant; DHPG,n=23, ***P=0.0001 compared with unstimulated conditions. (d) Histograms showing the mean±s.e.m. of the half-time constant in seconds computed for the exponential decay fit from independent synaptic Dendra2-Ubc9 photoconversion experiments. Pairedt-test: vehicle,n=21; DHPG,n=23, ***P=0.0001 compared with unstimulated (pre) conditions. (e) Scatter plots showing the mean±s.e.m. of half-time constant ratio of (post/pre) in control vehicle (1.001±0.025;n=21) and DHPG (1.824±0.156;n=23) conditions. Unpairedt-test; ***P=0.0001. Figure 4: mGlu5R activation promotes a transient diffusional trapping of Ubc9 in spines. ( a ) Time-lapse series of confocal images of photoconverted Dendra2-Ubc9 red fluorescence in spines in control and mGlu5R-stimulated conditions. Images of spine before Dendra2-Ubc9 photoconversion are shown in green (left). Following the first synaptic green-to-red photoconversion, neurons were incubated with control solution (vehicle) or with DHPG (50 μM) for 10 min and spines were photoconverted a second time. The red photoconverted fluorescence was then monitored as described in the Methods section. Scale bar, 1 μm. ( b ) Representative sample paired recording traces of normalized fluorescence from photoconverted Dendra2-Ubc9 in individual spines before (pre) and after mGlu5R activation (post) as shown in a . The thin traces (black) represent the corresponding fits. ( c ) Scatter plots of computed half-time of photoconverted Dendra2-Ubc9 fluorescence diffusion in spines pre- and post-DHPG application. Paired t -test: vehicle, n =21; NS, not significant; DHPG, n =23, *** P =0.0001 compared with unstimulated conditions. ( d ) Histograms showing the mean±s.e.m. of the half-time constant in seconds computed for the exponential decay fit from independent synaptic Dendra2-Ubc9 photoconversion experiments. Paired t -test: vehicle, n =21; DHPG, n =23, *** P =0.0001 compared with unstimulated (pre) conditions. ( e ) Scatter plots showing the mean±s.e.m. of half-time constant ratio of (post/pre) in control vehicle (1.001±0.025; n =21) and DHPG (1.824±0.156; n =23) conditions. Unpaired t -test; *** P =0.0001. Full size image Ca 2+ and PKC-dependent synaptic diffusional trapping of Ubc9 Our data indicate that mGlu5R activation regulates the diffusion of the SUMO-conjugating enzyme at hippocampal synapses. We therefore investigated the signalling pathways downstream of mGlu5R that could participate in this regulatory process ( Fig. 5 ). mGlu5R are coupled to Gα i and Gα q proteins [30] , [31] . Activation of Gα i downstream of mGlu5R stimulates cAMP-dependent protein kinase A (PKA) activity. To evaluate the involvement of this pathway on Ubc9 diffusion, we performed synaptic FRAP experiments in the presence of Pertussis toxin (PTX), a potent blocker of Gα i proteins [34] . We observed that the rate of GFP-Ubc9 fluorescence recovery as well as the diffusion coefficient values were unaffected by PTX, indicating that activation of Gα i proteins and the downstream activation of PKA is not required to regulate the synaptic diffusion of Ubc9 ( Fig. 5a–c ). 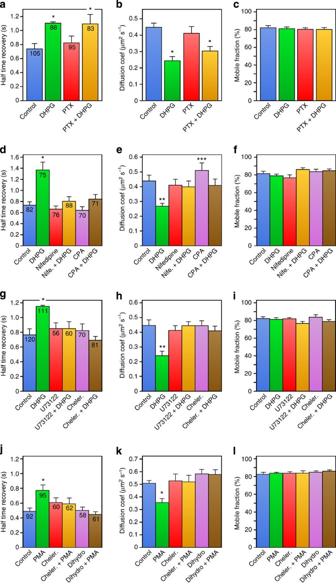Figure 5: The transient Ubc9 synaptic trapping involves PKC activation and requires Ca2+influx. Hippocampal neurons were treated with DHPG or not (Control) in the absence or in the presence of the Gαiblocker PTX (a–c), the voltage-dependent calcium channel (VDCC) blocker nifedipine (Nife.,d–f) or CPA, a potent inhibitor of the Ca2+-ATPase pumps (d–f), the PLC inhibitor U73122 (g–i) and the PKC inhibitor chelerythrine (Cheler.,g–i) as described in the Methods section. Neurons were treated with the phorbol ester PMA in the presence of selective PKC inhibitors, chelerythrine (Cheler.) or dihydrosphingosine (Dihydro). Histograms show the means (±s.e.m.) of half-time of recovery (a,d,g,j), diffusion coefficients (b,e,h,k) and mobile fractions (c,f,i,l) from the number of bleached spines indicated on the bars (a,d,g,j). One-way analysis of variance was performed with a Newman–Keuls post test for multiple comparison data sets. (a,b) *P<0.05 compared with Ctrl and PTX. (d) *P<0.001 compared with all treatments. (e) ***P=0.001 compared with DHPG and **P<0.01 compared with all treatments except CPA. (g) *P<0.01. (h) **P<0.001 compared with all treatments. (j,k) *P<0.01 PMA compared with all conditions. Mobile fractions (c,f,i,l) were not significantly different in all tested conditions. Figure 5: The transient Ubc9 synaptic trapping involves PKC activation and requires Ca 2+ influx. Hippocampal neurons were treated with DHPG or not (Control) in the absence or in the presence of the Gα i blocker PTX ( a – c ), the voltage-dependent calcium channel (VDCC) blocker nifedipine (Nife., d – f ) or CPA, a potent inhibitor of the Ca 2+ -ATPase pumps ( d – f ), the PLC inhibitor U73122 ( g – i ) and the PKC inhibitor chelerythrine (Cheler., g – i ) as described in the Methods section. Neurons were treated with the phorbol ester PMA in the presence of selective PKC inhibitors, chelerythrine (Cheler.) or dihydrosphingosine (Dihydro). Histograms show the means (±s.e.m.) of half-time of recovery ( a , d , g , j ), diffusion coefficients ( b , e , h , k ) and mobile fractions ( c , f , i , l ) from the number of bleached spines indicated on the bars ( a , d , g , j ). One-way analysis of variance was performed with a Newman–Keuls post test for multiple comparison data sets. ( a , b ) * P <0.05 compared with Ctrl and PTX. ( d ) * P <0.001 compared with all treatments. ( e ) *** P =0.001 compared with DHPG and ** P <0.01 compared with all treatments except CPA. ( g ) * P <0.01. ( h ) ** P <0.001 compared with all treatments. ( j , k ) * P <0.01 PMA compared with all conditions. Mobile fractions ( c , f , i , l ) were not significantly different in all tested conditions. Full size image mGlu5R are also coupled to the activation of Gα q proteins, which stimulate PLC, resulting in the formation of intracellular inositol-1,4,5-trisphosphate (IP3) and diacylglycerol. IP3 binding to its intracellular receptor leads to the release of Ca 2+ from internal stores, and together with diacylglycerol they activate PKC [30] , [31] . We first assessed the contribution of internal Ca 2+ stores to the regulation of Ubc9 diffusion in mGlu5R-activated spines by preincubating neurons with the potent inhibitor of the endoplasmic reticulum (ER) Ca 2+ -ATPase pump, the cyclopiazonic acid (CPA) [35] ( Fig. 5d–f ). We verified the effect of CPA using calcium imaging ( Supplementary Fig. 4 ) and then incubated GFP-Ubc9-expressing neurons in extracellular Ca 2+ -free medium to deplete internal Ca 2+ stores before DHPG activation in a CPA and Ca 2+ -containing buffer. Under these conditions, the mobile fractions remained unchanged by the pharmacological inhibition ( Fig. 5f ). Preincubation of neurons with CPA totally prevented the synaptic trapping of GFP-Ubc9 induced by DHPG ( Fig. 5d,e ; DHPG, 1.35±0.15 s; DHPG+CPA, 0.81±0.08 s, means±s.e.m.). In addition to the Ca 2+ rise from internal store that occurs in mGlu5R-stimulated cells, mGlu5R activation induces Ca 2+ influx through L-VDCC [30] , [31] . We therefore asked whether Ca 2+ influx through L-VDCC could also contribute to the regulation of Ubc9 diffusion in spines. We used the L-type Ca 2+ channel blocker Nifedipine [36] ; Supplementary Fig. 4 ) to inhibit Ca 2+ entry through L-VDCC following mGlu5R activation ( Fig. 5d–f ). DHPG application resulted in a significant increase in the half-time of GFP-Ubc9 fluorescence recovery ( Fig. 5d ; Control, 0.73±0.07 s; DHPG, 1.35±0.15 s, means±s.e.m.) and this effect was totally abolished when GFP-Ubc9-transfected neurons were co-incubated with Nifedipine (DHPG, 1.35±0.15 s; DHPG+Nife, 0.81±0.08 s, means±s.e.m.). Similar results were obtained for the diffusion coefficient values ( Fig. 5e ; DHPG, 0.44±0.04 μm 2 s −1 ; DHPG+Nife, 0.28±0.03 μm 2 s −1 , means±s.e.m. ), indicating that the Ca 2+ rise through L-VDCC in mGlu5R-stimulated neurons is required to regulate the synaptic mobility of Ubc9. These findings reveal a central role for Ca 2+ ions from external and internal sources in the regulation of Ubc9 diffusion in activated spines. We next assessed the involvement of the PLC/PKC signalling module downstream of mGlu5R in the regulation of Ubc9 diffusion in spines ( Fig. 5g–i ). We first incubated GFP-Ubc9-expressing neurons with the potent PLC antagonist U73122 (ref. 37 ) and performed FRAP to measure the synaptic properties of Ubc9 diffusion. Inhibiting PLC with U73122 occluded the effect of DHPG on the rate of GFP-Ubc9 fluorescence recovery ( Fig. 5g ; Control, 0.75±0.07 s; DHPG, 1.14±0.02 s, means±s.e.m.) without any significant modulation of the mobile fraction ( Fig. 5i ). Accordingly, the diffusion coefficient in DHPG-stimulated neurons in the presence of U73122 were not different from control conditions, indicating that PLC activation is necessary to regulate the mobility of Ubc9 in spines ( Fig. 5h ). We finally evaluated the involvement of PKC activity on the synaptic diffusion of Ubc9. We first blocked PKC activation using the cell-permeable inhibitor chelerythrine ( Fig. 5g–l ), which specifically binds to the catalytic domain of the kinase [38] . Incubation of GFP-Ubc9-transfected neurons with chelerythrine before mGlu5R activation fully abolished the mGlu5R-dependent increase in synaptic Ubc9 residency time evoked by DHPG ( Fig. 5g,h ; rates of recovery: DHPG, 1.14±0.02 s; DHPG+Cheler, 0.67±0.05 s; Diffusion coefficients: DHPG, 0.24±0.03 μm 2 s −1 ; DHPG+Cheler, 0.41±0.03 μm 2 s −1 , means±s.e.m. ), therefore indicating that PKC activation is involved in the regulation of Ubc9 diffusion in mGlu5R-activated neurons. To go further into the molecular mechanisms underlying the role of PKC in the regulation of Ubc9 diffusion, we incubated GFP-Ubc9-expressing neurons directly with the phorbol ester PMA [39] to activate PKC ( Fig. 5j–l ). PMA incubation led to synaptic FRAP parameters that were similar to those measured in DHPG-treated neurons with a significant increase in the half-time of GFP-Ubc9 fluorescence recovery ( Fig. 5j and Supplementary Fig. 5a,b ) and the concomitant decrease of Ubc9 diffusion coefficient in PMA-treated cells ( Fig. 5k ). Importantly, the PMA-induced Ubc9 trapping in spine was totally abolished when neurons were co-incubated with either the cell-permeable PKC inhibitor chelerythrine or the potent PKC blocker dihydrosphingosine [40] ( Fig. 5j,k and Supplementary Fig. 5a,b ). We then showed using synaptic photoconversion of Dendra2-Ubc9 in paired recordings that PKC activation with PMA led to a significant delay in the synaptic exit rate of the red photoconverted Dendra2-Ubc9 fluorescence ( Supplementary Fig. 5c–f ), further indicating that PKC activation is essential to promote the transient diffusional trapping of Ubc9 in mGlu5R-activated spines. mGlu5R- and PKC-dependent regulation of synaptic sumoylation Our data suggest that activation of mGlu5R triggers a PKC-dependent diffusional trapping of Ubc9 into spines that may lead to changes in synaptic sumoylation levels. To assess the direct impact of mGlu5R activation on synaptic sumoylation levels, we prepared synaptoneurosomes from P7 rat brains and pharmacologically stimulated in vitro these preparations before SUMO immunoblotting ( Fig. 6 ). Activation of mGlu5R using DHPG evoked an overall increase in synaptic sumoylation. Interestingly, there was a marked increase in synaptic SUMO1 sumoylation (DHPG, 145% of control) that was fully blocked in the presence of the specific mGlu5R antagonist MPEP ( Fig. 6a,b ) or using the PKC inhibitor chelerythrin. The direct activation of PKC with PMA also promoted a significant increase in synaptic SUMO1 immunoreactivity (PMA, 144% of control) that was fully prevented when neurons were co-incubated with chelerythrine. We were unable to detect free SUMO1 in synaptoneurosomes ( Fig. 6c ). However, as previously demonstrated [26] , [27] , the unmodified Ubc9 enzyme was slightly detectable in P7 rat synaptoneurosomes, whereas its SUMO1-modified form represented the main form of the enzyme and may therefore constitute a pool of SUMO1 directly available for conjugation ( Fig. 6a ). Free SUMO2 and SUMO2-modified protein levels remained unchanged throughout the experiments, although a slight increase was measured in the levels of SUMO2-modified proteins following stimulation with either DHPG or PMA ( Fig. 6a,b ). 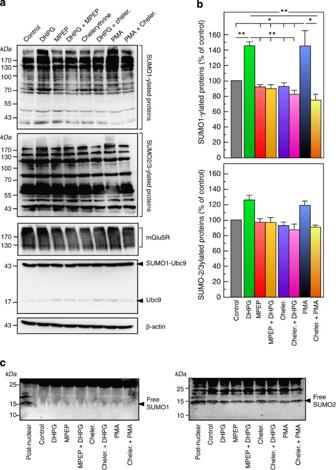Figure 6: mGlu5R activation leads to a PKC-dependent increase in synaptic sumoylation. (a) Representative immunoblottings showing immunoreactivities of synaptic sumoylated proteins, mGlu5R, SUMO1-Ubc9 and Ubc9 in basal and activated synaptosomes (n=5). Control β-actin was used as a loading control. (b) Summary histograms show means±s.e.m. of five independent experiments. One-way analysis of variance was performed with a Newman–Keuls post test. **P<0.001; *P<0.01. (c) Representative immunoblottings showing immunoreactivities of free SUMO moieties in basal and stimulated synaptosomes. Post-nuclear fractions obtained from P7 rat brain were used as a control (first lane) to show that free SUMO1 is detectable in our brain extracts but not in synaptosomes. Figure 6: mGlu5R activation leads to a PKC-dependent increase in synaptic sumoylation. ( a ) Representative immunoblottings showing immunoreactivities of synaptic sumoylated proteins, mGlu5R, SUMO1-Ubc9 and Ubc9 in basal and activated synaptosomes ( n =5). Control β-actin was used as a loading control. ( b ) Summary histograms show means±s.e.m. of five independent experiments. One-way analysis of variance was performed with a Newman–Keuls post test. ** P <0.001; * P <0.01. ( c ) Representative immunoblottings showing immunoreactivities of free SUMO moieties in basal and stimulated synaptosomes. Post-nuclear fractions obtained from P7 rat brain were used as a control (first lane) to show that free SUMO1 is detectable in our brain extracts but not in synaptosomes. Full size image Our data indicate that activation of mGlu5R promotes synaptic sumoylation through a PKC-dependent pathway. However, we showed that mGlu5R stimulation ( Fig. 4 ) or direct activation of PKC ( Supplementary Fig. 5c,f ) promotes a decrease in the exit rate of Ubc9 from spines. As synaptoneurosomes is a closed system, it suggests that the synaptic PKC-dependent SUMO conjugation is not directly due to the modulation of Ubc9 synapto-dendritic mobility, but rather results from an increased recognition of Ubc9 to PKC-phosphorylated substrates. The direct consequence of this increased recognition process in neurons would therefore be a transient diffusional trapping of Ubc9 in activated spines. Synaptic Ubc9 trapping implies a functional catalytic domain To validate our hypothesis that the synaptic diffusional trapping of Ubc9 results from an increased recognition of target proteins in activated neurons, we investigated the synaptic diffusion properties of the catalytically inactive and substrate-binding-deficient Ubc9-C93S mutant. Indeed, substrate recognition and enzymatic activity of Ubc9 are tightly linked, as its catalytic domain is essential for both processes [41] , [42] , [43] . It was shown that the cysteine residue in position 93 in Ubc9 forms the catalytic domain holding the SUMO moiety via a thioester bond before its catalytic transfer onto a specific lysine residue of a target protein. Therefore, Ubc9 binds directly to consensus sumoylation sequences of target proteins via its catalytic domain in a way that aligns the active C93-containing site directly next to the lysine residue to modify [42] . Importantly, the C93S substitution totally prevents sumoylation [42] , [43] , [44] . To assess whether the substrate recognition/catalytic activity of Ubc9 could be important for its synaptic regulation, we analysed the diffusion properties of the WT-active and the inactive GFP-Ubc9-C93S in mGlu5R-activated spines ( Fig. 7a–d ). We first ruled out potential side effects of the inactive form of GFP-Ubc9 on mGlu5R signalling pathway by investigating the levels of mitogen-activated protein kinase phosphorylation in response to DHPG [31] , in neurons expressing the active or inactive form of Ubc9. DHPG stimulation robustly induced Erk phosphorylation and this was not prevented on GFP-Ubc9-C93S mutant expression ( Fig. 7e ), indicating that the inactive Ubc9 does not occlude the downstream signalling of mGlu5R. 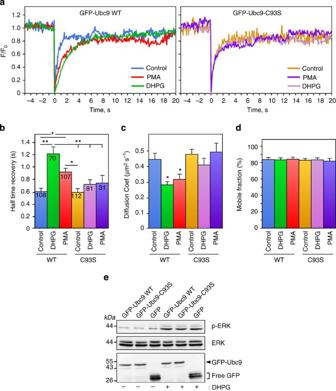Figure 7: The integrity of the catalytic domain of Ubc9 is crucial for the regulation of Ubc9 diffusion in spines. (a) Neurons expressing GFP-Ubc9 or its inactive C93S form were treated or not with DHPG or PMA. Normalized FRAP curves from individual spine showing recovery of WT and C93S GFP-Ubc9 fluorescence after photobleaching over the time course of the experiment. Summary histograms of FRAP experiments showing the means (±s.e.m.) of half-time of fluorescence recovery (b, **P<0.001 compared with all treatments except PMA; *P<0.05 compared with controls), diffusion coefficients (c, *P<0.01 DHPG, PMA compared with all treatments) and mobile fractions (d) from the number of bleached spines indicated on the bars (b). One-way analysis of variance with a Newman–Keuls post test. (e) Immunoblottings using anti-phospho- and total ERK antibodies of total proteins extracted from hippocampal neurons expressing the WT, the inactive C93S form of GFP-Ubc9 or free GFP as a control. Cells were treated or not for 10 min with DHPG. Note that the C93S mutation does not affect the DHPG-induced mGluR5 downstream signalling. The lower panel shows immunoblotting with anti-GFP antibodies to control for WT, mutant GFP-Ubc9 and free GFP protein levels. Figure 7: The integrity of the catalytic domain of Ubc9 is crucial for the regulation of Ubc9 diffusion in spines. ( a ) Neurons expressing GFP-Ubc9 or its inactive C93S form were treated or not with DHPG or PMA. Normalized FRAP curves from individual spine showing recovery of WT and C93S GFP-Ubc9 fluorescence after photobleaching over the time course of the experiment. Summary histograms of FRAP experiments showing the means (±s.e.m.) of half-time of fluorescence recovery ( b , ** P <0.001 compared with all treatments except PMA; * P <0.05 compared with controls), diffusion coefficients ( c , * P <0.01 DHPG, PMA compared with all treatments) and mobile fractions ( d ) from the number of bleached spines indicated on the bars ( b ). One-way analysis of variance with a Newman–Keuls post test. ( e ) Immunoblottings using anti-phospho- and total ERK antibodies of total proteins extracted from hippocampal neurons expressing the WT, the inactive C93S form of GFP-Ubc9 or free GFP as a control. Cells were treated or not for 10 min with DHPG. Note that the C93S mutation does not affect the DHPG-induced mGluR5 downstream signalling. The lower panel shows immunoblotting with anti-GFP antibodies to control for WT, mutant GFP-Ubc9 and free GFP protein levels. Full size image We then performed FRAP experiments on spines from WT and Ubc9-C93S-expressing neurons, and compared their diffusion properties ( Fig. 7a–d ). Mobile fractions remained unaffected by the C93S mutation ( Fig. 7d ). As expected, DHPG induced an increase in the half-time of fluorescence recovery for the WT Ubc9, while there was no difference when the inactive C93S mutant was analysed ( Fig. 7a,b ). These data were confirmed by comparing the diffusion coefficients where a significant drop was measured only in DHPG-treated cells expressing GFP-Ubc9 but not with its inactive C93S mutant ( Fig. 7c ; Control WT, 0.44±0.04 μm 2 s −1 ; DHPG WT, 0.28±0.03 μm 2 s −1 ; and DHPG WT versus DHPG C93S, 0.41±0.04 μm 2 s −1 , means±s.e.m. ), indicating that the enzymatic activity and/or the substrate recognition is important for the synaptic regulation of Ubc9 diffusion. Interestingly, PKC activation with PMA had no effect on the diffusion of the C93S mutant ( Fig. 7a–d ), invalidating a direct effect of PKC on Ubc9. Our data rather support our initial hypothesis that the transient diffusional trapping of Ubc9 into activated spine is due to the preferential anchoring of Ubc9 to synaptic PKC-phosphorylated protein substrates. Ubc9-binding to phosphoproteins causes synaptic trapping Many synaptic proteins are phosphorylated by PKC following mGlu5R stimulation [31] and it is now clear that many SUMO targets carry a PDSM [9] . This motif regulates the phosphorylation-dependent sumoylation of multiple substrates, including heat-shock factors and myocyte enhancer factor 2 (refs 9 , 10 ). To reinforce our hypothesis that mGlu5R activation leads to an increased synaptic anchoring of Ubc9 to PKC-phosphorylated substrates, we used the well-described PDSM discrimination-deficient Ubc9-K65A mutant [10] . Importantly, Ubc9-K65A loses its ability to discriminate between PDSM phosphorylation statuses but presents the ability to equally sumoylate phosphorylated and non-phosphorylated proteins in vitro [10] . Ubc9-K65A presented a subcellular distribution similar to the WT enzyme ( Fig. 8a ). We confirmed that the Ubc9-K65A mutant is able to sumoylate proteins ( Fig. 8b ). We then compared the diffusion properties of GFP-Ubc9 with the PDSM discrimination-deficient Ubc9-K65A mutant in mGlu5R-activated spines ( Fig. 8c–g ). DHPG stimulation induced a significant increase in the half-time of fluorescence recovery for the WT Ubc9 ( Fig. 8d,e ; Control WT, 0.63±0.04s; DHPG WT, 1.19±0.12s, means±s.e.m. ), while there was no difference for the PDSM discrimination-deficient mutant ( Fig. 8e ). Accordingly, a significant drop in the diffusion coefficient was measured in DHPG-treated neurons expressing WT GFP-Ubc9 ( Fig. 8f ; Control WT, 0.36±0.02 μm 2 s −1 ; DHPG WT, 0.21±0.02 μm 2 s −1 , means±s.e.m.) but not when the PDSM discrimination-deficient K65A mutant was analysed. 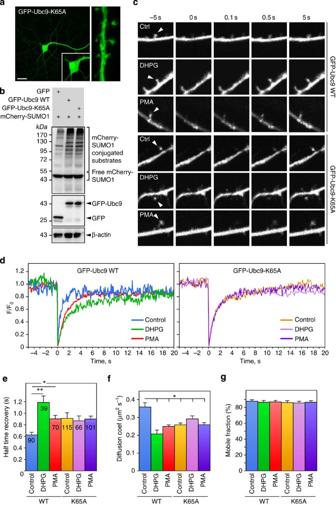Figure 8: Ubc9 trapping occurs via its recognition to PKC-phosphorylated proteins. (a) Representative image of a 20 DIV hippocampal neuron expressing the GFP-tagged PDSM discrimination-deficient Ubc9-K65A mutant. Insets show the nucleus and an enlarged dendrite. Scale bar, 20 μm. (b) Immunoblottings using anti-mCherry (top panel), anti-GFP (middle panel) or anti-β-actin antibodies (loading control) of total proteins extracted from COS7 cells expressing GFP-Ubc9, GFP-Ubc9-K65A mutant or free GFP together with mCherry-SUMO1. Molecular weight in kDa is shown. Sequential images (c) or normalized curves (d) from representative FRAP experiments on individual spine (arrowheads) from neurons expressing GFP-Ubc9 or GFP-Ubc9-K65A treated or not (Ctrl) with DHPG or PMA. Summary histograms of FRAP experiments showing the means (±s.e.m.) of half-time of fluorescence recovery (e, **P=0.001 and *P=0.01), diffusion coefficients (f, *P<0.01 compared with all conditions) and mobile fractions (g) from the number of bleached spines indicated on the bars (e). One-way analysis of variance with a Newman–Keuls post test. Figure 8: Ubc9 trapping occurs via its recognition to PKC-phosphorylated proteins. ( a ) Representative image of a 20 DIV hippocampal neuron expressing the GFP-tagged PDSM discrimination-deficient Ubc9-K65A mutant. Insets show the nucleus and an enlarged dendrite. Scale bar, 20 μm. ( b ) Immunoblottings using anti-mCherry (top panel), anti-GFP (middle panel) or anti-β-actin antibodies (loading control) of total proteins extracted from COS7 cells expressing GFP-Ubc9, GFP-Ubc9-K65A mutant or free GFP together with mCherry-SUMO1. Molecular weight in kDa is shown. Sequential images ( c ) or normalized curves ( d ) from representative FRAP experiments on individual spine (arrowheads) from neurons expressing GFP-Ubc9 or GFP-Ubc9-K65A treated or not (Ctrl) with DHPG or PMA. Summary histograms of FRAP experiments showing the means (±s.e.m.) of half-time of fluorescence recovery ( e , ** P =0.001 and * P =0.01), diffusion coefficients ( f , * P <0.01 compared with all conditions) and mobile fractions ( g ) from the number of bleached spines indicated on the bars ( e ). One-way analysis of variance with a Newman–Keuls post test. Full size image To further highlight the central role of PKC activity in the diffusional trapping of Ubc9 in activated spines, we compared the diffusion values measured from neurons expressing GFP-Ubc9 or its K65A mutant in the presence of the PKC activator PMA ( Fig. 8c–g ). Treating GFP-Ubc9-expressing neurons with PMA resulted in a significant increase in the half-time of fluorescence recovery and the concurrent decrease in the diffusion coefficient, whereas PKC activation had no effect on the synaptic mobility of the PDSM discrimination-deficient K65A mutant ( Fig. 8d–f ). To confirm the functional impact of a tightly controlled Ubc9 regulation in spines, we analysed the excitability of neurons expressing the PDSM discrimination-deficient K65A mutant ( Supplementary Fig. 6 ). We showed that the neuronal excitability measured for the K65A mutant is significantly decreased when compared with the WT enzyme. Indeed, although the resting potentials in WT and mutant conditions were almost similar ( Supplementary Fig. 6c ), the frequency of spontaneous action potentials in K65A-expressing neurons was significantly lower than in cells expressing the WT Ubc9 ( Supplementary Fig. 6a,b ; K65A, 0.49±0.11 Hz; WT, 1.05±0.20 Hz, means±s.e.m. ). Here we have investigated the regulatory mechanisms of Ubc9, the sole conjugating enzyme of the sumoylation system during the modulation of synaptic activity. Our work demonstrates that Ubc9 diffusion at hippocampal synapses is impacted by activity providing several important insights into the mechanisms that underlie this activity dependence ( Fig. 9 ). This regulation involves an mGlu5R-dependent signalling pathway. Neuronal activation using either the GABA A R antagonist bicuculline or the direct exposure of neurons to group I mGluR agonist increases the synaptic residency time of Ubc9 and this effect is blocked using the specific mGlu5R antagonist MPEP. The downstream mGlu5R-signalling pathway regulating the synaptic diffusion of Ubc9 involves a PLC/PKC activation cascade. Importantly, the direct PKC activation mimicked the effect of mGlu5R stimulation on Ubc9 diffusion, whereas blocking PKC activity abolished the diffusional trapping of Ubc9 in activated spines. Activation of mGlu5R promotes synaptic sumoylation through a PKC-dependent pathway, suggesting that Ubc9-driven SUMO conjugation results from an increased anchoring of Ubc9 to PKC-phosphorylated proteins. Consistently, the catalytic domain of Ubc9 comprising the C93 residue, known to be essential for the activity and substrate recognition of the enzyme [42] , [43] , [44] , is also central to the synaptic regulation of Ubc9 diffusion through the PKC-dependent phosphorylation of synaptic proteins. We confirmed this transient PKC-dependent anchoring of Ubc9 in activated spines using the phosphorylation discrimination-deficient Ubc9-K65A mutant and demonstrate its impact on neuronal excitability. 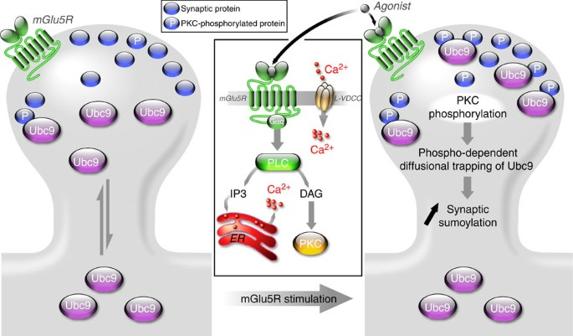Figure 9: Schematic model of the synaptic regulation of sumoylation.  Figure 9: Schematic model of the synaptic regulation of sumoylation. Full size image Our data also demonstrated that blocking the intracellular Ca 2+ rise through L-VDCC or the Ca 2+ release from internal ER store in mGlu5R-activated neurons abolished the synaptic regulation of Ubc9 diffusion. These results suggest that the Ca 2+ released from the ER is downstream of the VDCC-mediated Ca 2+ influx. This is consistent with recent data showing that large synaptic complexes comprising mGlu5R, IP3 receptors and L-VDCC play key roles in the calcium-current facilitation evoked by mGlu5R activation [45] . The mGlu5R-induced calcium-current facilitation requires the activation of calcium-induced calcium release that was triggered by the L-VDCC opening [45] . It was also reported using L-VDCC knockout mice that activation of mGlu5R sensitized both IP3 and ryanodin receptors onto the ER to Ca 2+ entry through the L-type voltage-gated Cav1.3 channels, and that this event promoted calcium-induced calcium release that was essential to promote synaptic plasticity [46] . It is therefore not surprising to see that the blockade of Ca 2+ influx from both L-VDCC and internal ER stores prevent the synaptic trapping of Ubc9 and reinforce our conclusion that a Ca 2+ rise is critical for the synaptic regulation of sumoylation. Another potential mechanism for the regulation of Ubc9 function could be the direct phosphorylation of the enzyme. It was reported that Ubc9 could be phosphorylated in vitro on serine 71 by the CDK1/cyclin B kinase but not by other kinases including PKA, ERK, JNK2 or CDK2. The direct effect of Ubc9 phosphorylation by CDK1 is an increased SUMO conjugation [47] . However, the authors cannot rule out the possibility that this increased sumoylation may also result from the CDK1-dependent phosphorylation of other proteins, thereby increasing Ubc9 binding/recognition and subsequently sumoylation of CDK1-phosphorylated substrates. Intriguingly, the Ubc9-K65A mutant showed diffusion parameters similar to those measured for the WT form of the enzyme in mGlu5R- or PMA-activated conditions. These results suggest that contrary to WT Ubc9, the K65A mutant is able to recognize and bind to additional non-phosphorylated synaptic substrates in resting conditions, leading to an apparent reduced diffusion in non-activated spines. As Ubc9-K65A is unable to discriminate the phosphorylation status of the substrates, it is not surprising that we cannot measure any additional diffusional trapping in mGlu5R or PMA-stimulated conditions. Moreover, the neuronal expression of the K65A mutant led to a decrease in neuronal excitability highlighting a functional role for the regulation of the sumoylation process in synaptic communication. The fact that neuronal excitability is decreased in PDSM discrimination-deficient Ubc9-expressing neurons will lead to many exciting research avenues, as numerous unidentified synaptic proteins may be targeted for sumoylation in a non-regulated manner. It also implies that the balance between sumoylation and desumoylation is impacted when the Ubc9-K65A mutant is expressed. Further work will now be required to identify synaptically activated sumoylation substrates and to characterize the regulatory mechanisms of desumoylation enzymes in spines. Interestingly, sumoylation of some synaptic proteins has already been shown to require phosphorylation before sumoylation. Konopacki et al . [23] reported the agonist-induced PKC phosphorylation of the kainate receptor GluK2 C-terminus and showed that this event is required for GluK2 sumoylation [23] . Both events were shown to be essential for the endocytosis of GluK2 that occurs during kainate receptor-mediated long term depression at hippocampal mossy fibre synapses [25] and are consistent with our work showing that the mGlu5R-driven synaptic phosphorylation triggers the binding of Ubc9 to de novo PKC-phosphorylated proteins and the transient synaptic trapping of Ubc9. Another interesting aspect of our work is that sumoylation can act as a ubiquitin antagonist by competing at specific lysine residues on target proteins to inhibit protein degradation [15] , [16] . For instance, Bingol and Schuman [29] demonstrated that the synaptic trafficking of the proteasome is activity regulated. Indeed, NMDAR activation induces the translocation of the proteasome into spines, leading to ubiquitination and degradation of synaptic proteins [29] . The direct consequence of this is the shaping of the synaptic protein content. Here we demonstrate that the synaptic regulation of Ubc9 does not involve NMDAR but mGlu5R. Our data therefore add an additional level of regulation in the control of the synaptic protein content, as these two post-translational modifications can target the same residue to regulate protein degradation. Our work also raises intriguing questions as to the role of sumoylation in brain disorders involving altered group I mGluR-signalling pathways. Indeed, these receptors have been involved in the modulation of synaptic transmission and plasticity [30] , [31] , and in the pathogenesis of various central nervous system disorders, including but not restricted to schizophrenia or chronic pain, as well as several neurological diseases [31] . We show that the synaptic diffusion of Ubc9 is regulated through an mGlu5R-dependent signalling pathway. Thus, under pathological conditions, the deregulated mGlu5R signalling could modify Ubc9 diffusion and consequently induce changes in protein sumoylation, leading to altered synaptic function. Therefore, an important focus of future studies will be to characterize sumoylation in brain disorders where mGlu5R signalling is deregulated. Constructs The Gateway destination vector for the fusion of open reading frames to the amino terminus of mouse Ubc9 sequence is a generous gift from Dr Niedenthal [48] . The GFP-Ubc9 construct was made by inserting the GFP coding sequence in frame with the N-terminus of Ubc9 with the Gateway recombination technology (Invitrogen). Ubc9-C93S and K65A mutant constructs were made by site-directed mutagenesis using Quick-change mutagenesis (Agilent). Cell culture Hippocampal neurons were prepared from E18 pregnant Wistar rats as previously described [27] , [49] . Briefly, cells were plated in Neurobasal medium (Invitrogen, France) supplemented with 2% B27 (Invitrogen), 0.5 mM glutamine and penicillin/streptomycin on 24-mm glass coverslips pre-coated with poly- L -lysine (0.1 mg ml −1 ). Neurons (110,000 cells per coverslip) were fed once a week for 3 weeks in Neurobasal medium supplemented with 2% B27 and penicillin/streptomycin. All procedures were approved by our local Animal Ethics Committee (Comité Institutionnel d’Éthique Pour l’Animal de Laboratoire N°28, Nice, France; Project reference NCE/2012-63). Neuronal transfection Hippocampal neurons (18–20 days in vitro (DIV)) were transfected using Lipofectamin 2000 (Invitrogen), according to the manufacturer’s instructions, with 3 μg of plasmid DNA and used 48–72 h post transfection. Immunocytochemistry Hippocampal neurons (19–21 DIV) treated or not for 10 min with 50 μM DHPG at 37 °C were fixed with paraformaldehyde 4% in PBS for 10 min at room temperature (RT) and washed three times for 5 min in PBS. Cells were then permeabilized for 20 min in PBS containing 0.1% Triton X-100 and 10% Horse Serum at RT. Neurons were immunostained with a mouse anti-Ubc9 (1/50; BD Bioscience, France) and a rabbit anti-Homer1 (1/200; Synaptic System, Germany) overnight at 4 °C in PBS containing 0.05% Triton X-100 and 5% HS. Cells were washed three times in PBS and incubated with the appropriate secondary antibodies conjugated to Alexa488 or Alexa594, and mounted with Mowiol (Sigma). Confocal images (1,024 × 1,024 pixels) were acquired with a × 63 oil-immersion lens (numerical aperture (NA) 1.4) on an inverted TCS-SP5 confocal microscope (Leica Microsystems, France). Z-series of seven to eight images of randomly selected dendrites were compressed into two dimensions using the maximum projection algorithm of the Leica software. Quantification was performed using ImageJ software and the synaptic enzymatic staining was measured with the use of an in-house ImageJ macro [26] , [27] . Briefly, confocal image of the synaptic marker was used to produce a mask after an automated intensity threshold. Masks were applied to the corresponding images, and the fluorescence intensity within the synaptic area was measured. Calcium imaging Hippocampal neurons were loaded in neurobasal containing 5 μM of Fura-2AM (Invitrogen) for 30 min and then washed and incubated for an additional 30 min period in neurobasal medium. After a further three washes in Earle’s buffer (25 mM HEPES-Tris pH 7.4, 140 mM NaCl, 5 mM KCl, 1.8 mM CaCl 2 , 0.8 mM MgCl 2 , 0.9 g l −1 glucose), Fura-2AM-loaded neurons were continuously perfused (1 ml min −1 , 37 °C) on an inverted microscope (AxioObserver, Carl Zeiss) equipped with a 300W Xenon lamp (Suttler Instruments) and a Fluar × 40 (NA 1.4) oil-immersion objective. Fura-2AM was sequentially excited at 340 and 380 nm and the emission monitored at 510 nm. Images were acquired with a cascade 512 EMCCD camera every 5 s and digitized using Metafluor software (Roper Scientific). The intracellular calcium concentration [Ca 2+ ]i was estimated by measuring the F340/380 nm fluorescence ratio. Neurons were treated with various pharmacological drugs: 50 μM DHPG, 50 μM MPEP, 10 μM Nifedipine or 20 μM CPA diluted in Earle’s buffer. Live cell imaging Protocols were performed as previously described [49] , [50] . Briefly, dendrites from live GFP- or GFP-Ubc9-transfected neurons (19–20 DIV) were kept on a heated stage (set at 37 °C) on a Nikon Ti inverted microscope. GFP fluorescence was excited through a × 100 oil-immersion lens (NA, 1.4) using a 488-nm laser light (50 mW, 1–2%) and time series (15 Hz) were collected for 25 s as a single image slice using a Perkin Elmer Ultra-View spinning disk solution. Neurons were treated or not with 10 μM bicuculline, 2 μM TTX or 50 μM DHPG in Earle’s buffer (25 mM HEPES-Tris pH 7.4, 140 mM NaCl, 5 mM KCl, 1.8 mM CaCl 2 , 0.8 mM MgCl 2 , 0.9 g l −1 glucose) for 10–20 min in Earle’s buffer. A 10–20 min preincubation at 37 °C was achieved when specific inhibitors were used. Pharmacological drugs (MPEP 30 μM, D-APV 50 μM, PTX 0.5 μg ml −1 , U73122 2 μM, chelerythrine 5 μM, dihydrosphingosine 50 μM, PMA 2 μM, nifedipine 10 μM or CPA 20 μM) were diluted in Earle’s buffer. FRAP measurements Fluorescence intensity variations in spines were analysed using the FRAP module of the Volocity 6.3 software. Fluorescence recovery curve in FRAP allows the direct determination of two parameters. First, the difference between the basal level of fluorescence and the recovered plateau level after photobleaching reflects the immobile fraction of protein and conversely the mobile diffusible fraction. Immobile fractions reflect the direct or indirect binding of the protein of interest to cytoskeleton constituents. Second, the half-time of recovery specifies the mobility of the diffusible fraction of the protein of interest. Fluorescence data were collected from regions of interest drawn around the fluorescence of GFP- or GFP-Ubc9-expressing spines or shafts. FRAP data were expressed as a percentage of initial fluorescence (average fluorescence value from the 5-s imaging period immediately before photobleaching) over time and fitted with a single-phase exponential function ( f(t) =y+A e−kt ) using the Volocity 6.3 software from Perkin Elmer. Mobile fraction (in %), half-time of recovery (in seconds) and diffusion coefficient (in μm 2 s −1 ; D =photobleached spine area/4 t 1/2 ) values were extracted for each experiment using the FRAP module of the Volocity 6.3 software. Dendra2-Ubc9 photoconversion measurements For Dendra2-Ubc9 experiments, the GFP tag from the GFP-Ubc9 construct was exchanged for the green-to-red photoswitchable Dendra2 protein [32] , [33] (Evrogen JSC, Russia). Individual Dendra2-Ubc9-expressing spines were photoconverted for 30 ms using a 405-nm laser light (50 mW, 100%). The red photoconverted Dendra2-Ubc9 was excited using a 561-nm laser light (50 mW, 20%) and time series (10 Hz) were collected for 20 s as a single image slice using a Perkin Elmer Ultra-View spinning disk solution. For paired recordings of synaptic Dendra2-Ubc9 photoconversion, spines were first photoconverted and imaged for 20 s followed by a 10-min period in either control (vehicle) or the indicated drug solution at 37 °C and then photoconverted/imaged a second time. The decrease in red fluorescence from the Dendra2-Ubc9 photoconverted spines was measured over time using the Volocity 6.3 software and data expressed as a percentage of the initial red photoconverted fluorescence ( F / F 0 ). Curves were fitted using a mono-exponential decay equation and data statistically analysed (paired and unpaired t -test as indicated) with Prism 4 (GraphPad software, Inc). Synaptosomal preparation and stimulation Brains (12 Wistar P7 rats) were homogenized at 4 °C in 7 volumes (w/v) of 10 mM Tris buffer (pH 7.4) containing 0.32 M sucrose and protease inhibitors (Complete EDTA-free; Roche, USA) [51] , [52] . The resulting homogenate was centrifuged at 1,000 g for 5 min at 4 °C to remove nuclei and cellular debris. Synaptosomal fractions were purified by centrifugation for 10 min at 14,000 r.p.m. (SW41Ti rotor) at 4 °C using Percoll-sucrose density gradients (2-6-10-20%; v/v). Each fraction from the 10–20% interface was collected, washed in 10 ml of a 5 mM HEPES buffer pH 7.4 (NaOH) containing 140 mM NaCl, 3 mM KCl, 1.2 mM MgSO 4 , 1.2 mM CaCl 2 , 1 mM NaH 2 PO 4 , 5 mM NaHCO 3 , 10 mM glucose by centrifugation. Synaptosomes were resuspended in 0.6 ml of the same buffer at RT and gently agitated at 37 °C. After 10 min, antagonists, inhibitors or vehicle were added to synaptosomes for 10 min before synaptosomal stimulation with the indicated drug for a further 10 min at 37 °C. Ice-cold HEPES medium (0.6 ml) containing freshly prepared NEM (40 mM) was then added to the stimulated synaptosomes and the suspension was immediately centrifuged at 10,000 g at 4 °C for 5 min. Pellets were resuspended in 2 × Laemlli buffer containing 5% βME, boiled for 10 min and analysed by immunoblotting. Intensities of bands on the immunoblottings were quantified using Bio1D software (Vilber-Lourmat, France). Densitometric values measured from each lane were compared with the corresponding untreated control fraction. Immunoblotting Transfected COS7 cells (ATCC, Molsheim, France) were homogenized in lysis buffer (10 mM Tris–HCl pH7.5, 10 mM EDTA, 150 mM NaCl, 1% Triton X100, 0.1% SDS) in the presence of a mammalian protease inhibitor cocktail (Sigma, 1/100) and 20 mM freshly prepared NEM (Sigma) to protect proteins from desumoylation. Protein extracts (30 μg) were resolved by SDS–PAGE and immunoblotted with primary antibodies: rabbit polyclonal anti-SUMO1 (ref. 53 ), 1.7 μg ml −1 ; rabbit anti-SUMO2/3 (ref. 27 ), 1/240; Invitrogen, USA; mouse anti-Ubc9 (refs 20 , 26 ), 1/200, BD Bioscience, France; mouse anti-GFP, 1/1,000, Roche, Germany, or rat anti-mCherry [54] , 1/500, ChromoTek GmbH, Germany; mouse anti-phosphorylated-ERK and rabbit anti-ERK [55] , 1/1,000, Tebu-Bio, France. Standard β-actin loading controls were included using a mouse anti-β-actin antibody (1/5,000, Sigma). Full-size blottings for cropped gels can be found in Supplementary Fig. 7 . Electrophysiological recordings Neuronal excitability of transfected neurons (19–21 DIV) was assessed using whole-cell configuration of the patch clamp technique. Membrane potentials were recorded for 3 min at RT using an axopatch 200B amplifier (Axon Instruments) with a 2-kHz low-pass filter. Data were sampled at 10 kHz, digitized by a Digidata 1440 A-D/D-A converter (Axon Instruments), recorded and analysed using pClamp software. Patch pipettes (3–6 MΩ) contained (in mM): 135 KCl, 2.5 Na 2 -ATP, 2 MgCl 2 , 2.1 CaCl 2 , 5 EGTA, 10 HEPES (pH 7.25 with KOH). Control bath solution contained (in mM): 145 NaCl, 5 KCl, 2 MgCl 2 , 2 CaCl 2 , 10 HEPES, 10 glucose (pH 7.4 with NaOH). Statistical analysis Statistical analyses were calculated using GraphPad Prism 4 (GraphPad software, Inc.). Data were expressed as mean±s.e.m. One-way analysis of variance were performed with a Newman–Keuls post test for multiple comparison data sets. All data were tested for normal distribution. Statistical analyses for electrophysiological data were computed using a Mann–Whitney test. How to cite this article: Loriol, C. et al . mGlu5 receptors regulate synaptic sumoylation via a transient PKC-dependent diffusional trapping of Ubc9 into spines. Nat. Commun. 5:5113 doi: 10.1038/ncomms6113 (2014).